Hepatic miR-378 targets p110α and controls glucose and lipid homeostasis by modulating hepatic insulin signalling Understanding the regulation of insulin signalling in tissues provides insights into carbohydrate and lipid metabolism in physiology and disease. Here we show that hepatic miR-378/378* expression changes in response to fasting and refeeding in mice. Mice overexpressing hepatic miR-378/378* exhibit pure hepatic insulin resistance. miR-378 inhibits hepatic insulin signalling through targeting p110α, a subunit of PI3K and hence a critical component of insulin signalling. Knockdown of hepatic p110α mimics the effect of miR-378, while restoration of p110α expression abolishes the action of miR-378 on insulin signalling as well as its systemic effects on glucose and lipid homeostasis. miR-378/378* knockout mice display hypoglycemia and increased hepatic triglyceride level with enhanced insulin sensitivity. Inhibition of hepatic p110α in miR-378/378* knockout mice corrects the abnormal glucose tolerance. Finally, we show that overexpression of hepatic miR-378/378* ameliorates hepatic steatosis in ob/ob mice without exacerbating hyperglycemia. Our findings establish fasting-responsive miR-378 as a critical regulator of hepatic insulin signalling. The liver is a metabolic organ that senses and integrates multiple signals delivered via hormones, neuronal impulses and metabolic and nutritional factors. It plays important roles in controlling glucose and lipid homeostasis to meet energy needs in response to different metabolic stresses [1] , [2] , [3] . Insulin is critical for both carbohydrate and lipid metabolism. During the transition from a fasted state to a fed state, increased blood sugar level triggers the secretion of insulin, which will suppress gluconeogenesis, stimulate glycogen synthesis and activate lipogenesis in the liver [4] , [5] . Hepatic insulin resistance is a critical component in the development of metabolic diseases, such as type 2 diabetes mellitus. In the state of insulin resistance, the effect of insulin is repressed and the persistence of hepatic glucose output contributes to the postprandial hyperglycemia [6] , [7] . Studies on the complex network of hepatic insulin signalling should help to understand the molecular mechanisms underlying hepatic insulin resistance and provide new strategies for treating metabolic disorder. Phosphoinositide 3-kinase (PI3K) heterodimer together with insulin receptor/insulin-receptor substrate (IR/IRS) and serine–threonine protein kinase (Akt/PKB) are the three best-defined and critical nodes of the insulin signalling pathway [8] . Many effects of insulin on metabolism have been attributed to the signalling through PI3K. PI3K consists of a regulatory subunit (p85) and a catalytic subunit (p110). It has been demonstrated that p110α plays a fundamental role in hepatic insulin/PI3K signalling and controls glucose and lipid homeostasis. In response to feeding, activation of PI3K by insulin in the liver leads to phosphorylation of Akt at residues Thr 308 and Ser 473, and the activated Akt in turn inhibits gluconeogenesis and stimulates glycogen synthesis through inactivation of forkhead box O1 (FOXO1) and glycogen synthase kinase 3β (GSK3β) via phosphorylation. Meanwhile, activated PI3K is capable of enhancing hepatic lipogenesis through Akt or protein kinase Cλ [9] , [10] , [11] , [12] . In contrast, in response to food deprivation, insulin/PI3K signalling is less active to ensure that glucose production is not repressed. As PI3K heterodimer is a critical node of insulin signalling in the liver, the regulatory role of PI3K has been investigated extensively. However, little is known about the regulation of PI3K expression at posttranscriptional level. MicroRNAs (miRNAs) are small non-coding RNAs (~22 nucleotides) that regulate target gene expression posttranscriptionally. It has been shown that miRNA could represent another crucial regulatory layer in regulating insulin action [13] , [14] . miR-103/107 and let-7 mainly regulate insulin signalling in peripheral tissues such as adipose tissue and skeletal muscle by targeting caveolin-1 and IR/IRS2 , respectively [15] , [16] . miR-143 and miR-34a affect hepatic insulin signalling by targeting oxysterol-binding-protein-related protein 8 ( ORP8 ) and Sirtuin 1 ( SIRT1 ), respectively [17] , [18] . miR-33 affects hepatic insulin action by targeting multiple metabolic regulators, including Sirtuin 6 ( SIRT6 ), α1 subunit of AMP-activated protein kinase ( AMPKα1 ) and IRS2 . However, whether one of these metabolic regulators alone or all of them contribute to the regulatory role of miR-33 on insulin signalling remains unclear [19] . miR-378 and miR-378* , which are derived from a common hairpin RNA precursor, are located in the first intron of peroxisome proliferator-activated receptor γ coactivator-1β ( PGC-1β ) [20] . Mice genetically lacking miR-378/378* are resistant to high-fat diet-induced obesity and exhibit enhanced mitochondrial fatty acid metabolism, suggesting that miR-378/378* might be involved in the regulation of mitochondrial metabolism and systemic energy homeostasis [21] . In breast cancer, miR-378* upregulation results in an increase in cell proliferation and lactate production, and a repression of tricarboxylic acid cycle and oxygen consumption, indicating that miR-378* is able to mediate metabolic shift in cancer cells [20] . It has also been reported that hepatic miR-378/378* expression is dysregulated in a rat model of type 2 diabetes and obese mouse models, including genetic ob/ob mice and mice fed a high-fat diet [15] , [21] , [22] . However, whether and how miR-378 or miR-378* plays a regulatory role in hepatic glucose and lipid metabolism remains unclear. Here we report that mice overexpressing hepatic miR-378/378* share many phenotypic features of those mice deficient in key components of insulin signalling, such as insulin receptor [23] , [24] , p110α [25] , [26] , [27] , p85 (ref. 28 ) and Akt2 (refs 29 , 30 ), while miR-378/378* knockout (378KO) mice display fasting hypoglycemia and increased hepatic triglyceride level with enhanced insulin sensitivity. We also demonstrate that miR-378 inhibits insulin signalling through targeting p110α, and increasing hepatic miR-378/378* levels in ob/ob mice ameliorates hepatic steatosis without exacerbating fasting hyperglycemia. These findings let us to propose that fasting-responsive hepatic miR-378 is a critical regulator of glucose and lipid homeostasis, and may serve as a potential therapeutic target for metabolic diseases. Hepatic miR-378/378* regulates glucose homeostasis To see whether miR-378/378* is involved in the regulation of hepatic metabolism, we first determined the expression levels of miR-378 and miR-378* in the liver of C57BL/6J mice under different feeding conditions. As shown in Fig. 1a and Supplementary Fig. 1a,b , both miR-378 and miR-378* expression levels were elevated during fasting and were repressed after refeeding. The expression pattern of miR-378/378* was similar to the pattern of its host gene PGC-1β and gluconeogenic genes, phosphoenolpyruvate carboxykinase ( PEPCK ) and glucose-6-phosphatase ( G6Pase ) ( Supplementary Fig. 1c,d ). In contrast, the expression pattern of miR-378/378* was opposite to the pattern of lipogenic genes, acetyl-CoA carboxylase ( ACC1 ) and fatty acid synthase ( FASN ) ( Supplementary Fig. 1e ). These data suggested that hepatic miR-378/378* might be involved in glucose and lipid metabolism during the fasting–refeeding transition. 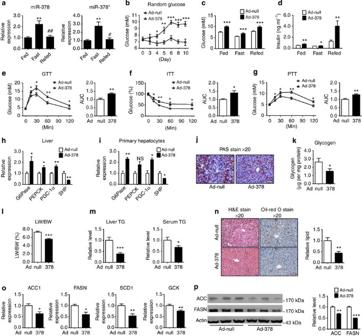Figure 1: miR-378/378* overexpression dysregulates glucose/lipid homeostasis. (a) The levels of miR-378/378* in the liver of fed, fasted and refed mice (n=5). Means±s.e.m. are shown. **P<0.01 versus fed mice;#P<0.05 versus fasted mice;##P<0.01 versus fasted mice. (b) Time course of random glucose levels of mice after Ad-null or Ad-378 infection (n=9-10). Blood glucose levels (c,n=15–17) and insulin levels (d,n=8–9) of mice infected with Ad-null or Ad-378 were examined under different feeding conditions. (e–g) Glucose-tolerance test (GTT;e,n=6–7), insulin-tolerance test (ITT;f,n=9–10) and pyruvate-tolerance test (PTT) (g,n=9–10) were performed in mice infected with Ad-null or Ad-378. Area under the curve (AUC) data for GTT (e), ITT (f) and PTT (g) tests were calculated, respectively. The expression ofG6Pase,PEPCK,PGC-1αandSHPin the liver of mice (h,n=5) or mouse primary hepatocytes (i,n=3) infected with Ad-null or Ad-378 as indicated. PAS staining (j) and glycogen assay (k,n=7) were carried out to determine the glycogen storage in the liver of mice infected with Ad-null or Ad-378. Representative results of PAS staining were shown (j). Scale bar, 50 μm. The amount of glycogen was normalized based on protein weight (k). (l) The ratio of liver weight to body weight (LW/BW) was determined in mice infected with Ad-null or Ad-378 (n=10-11). (m) Liver and serum TG levels were measured in random fed state (n=10-11). (n) Representative images of H&E staining (left) and Oil-red O staining (right) of liver sections fromad libitum-fed mice infected with Ad-null (top) or Ad-378 (bottom). Scale bar, 50 μm. Image-Pro Plus was employed for quantification of lipid content. (o) Relative mRNA levels ofACC1,FASN,SCD1andGCKin the liver of mice infected with Ad-null or Ad-378 (n=5). (p) Protein levels of ACC and FSAN were determined by western blot analysis and quantified. Each mouse received 1 × 109PFU of adenovirus. Means±s.e.m. are shown for all panels. *P<0.05 versus control; **P<0.01 versus control; ***P<0.001 versus control (Student’st-test). All experiments were repeated at least twice and representative results are shown. Figure 1: miR-378/378* overexpression dysregulates glucose/lipid homeostasis. ( a ) The levels of miR-378/378* in the liver of fed, fasted and refed mice ( n =5). Means±s.e.m. are shown. ** P <0.01 versus fed mice; # P <0.05 versus fasted mice; ## P <0.01 versus fasted mice. ( b ) Time course of random glucose levels of mice after Ad-null or Ad-378 infection ( n =9-10). Blood glucose levels ( c , n =15–17) and insulin levels ( d , n =8–9) of mice infected with Ad-null or Ad-378 were examined under different feeding conditions. ( e – g ) Glucose-tolerance test (GTT; e , n =6–7), insulin-tolerance test (ITT; f , n =9–10) and pyruvate-tolerance test (PTT) ( g , n =9–10) were performed in mice infected with Ad-null or Ad-378. Area under the curve (AUC) data for GTT ( e ), ITT ( f ) and PTT ( g ) tests were calculated, respectively. The expression of G6Pase , PEPCK , PGC-1α and SHP in the liver of mice ( h , n =5) or mouse primary hepatocytes ( i , n =3) infected with Ad-null or Ad-378 as indicated. PAS staining ( j ) and glycogen assay ( k , n =7) were carried out to determine the glycogen storage in the liver of mice infected with Ad-null or Ad-378. Representative results of PAS staining were shown ( j ). Scale bar, 50 μm. The amount of glycogen was normalized based on protein weight ( k ). ( l ) The ratio of liver weight to body weight (LW/BW) was determined in mice infected with Ad-null or Ad-378 ( n =10-11). ( m ) Liver and serum TG levels were measured in random fed state ( n =10-11). ( n ) Representative images of H&E staining (left) and Oil-red O staining (right) of liver sections from ad libitum -fed mice infected with Ad-null (top) or Ad-378 (bottom). Scale bar, 50 μm. Image-Pro Plus was employed for quantification of lipid content. ( o ) Relative mRNA levels of ACC1 , FASN , SCD1 and GCK in the liver of mice infected with Ad-null or Ad-378 ( n =5). ( p ) Protein levels of ACC and FSAN were determined by western blot analysis and quantified. Each mouse received 1 × 10 9 PFU of adenovirus. Means±s.e.m. are shown for all panels. * P <0.05 versus control; ** P <0.01 versus control; *** P <0.001 versus control (Student’s t -test). All experiments were repeated at least twice and representative results are shown. Full size image To explore the function of hepatic miR-378/378* in vivo , adenoviral miR-378/378* (Ad-378) (1 × 10 9 plaque-forming unit (PFU)) was used to achieve overexpression of miR-378/378* in the liver of mice ( Supplementary Fig. 1f ). Interestingly, we found that glucose levels of mice fed ad libitum were increased gradually after injection of 1 × 10 9 PFU of Ad-378 ( Fig. 1b ). Moreover, the elevated glucose levels were also observed in these mice overexpressing miR-378/378* under other feeding conditions ( Fig. 1c ). Concomitant with the increased glucose levels, insulin levels were also elevated in these mice ( Fig. 1d ). Furthermore, hepatic overexpression of miR-378/378* resulted in impaired glucose tolerance and insulin tolerance ( Fig. 1e,f ). These results indicated that hepatic miR-378/378* is able to affect glucose homeostasis. The observation above prompted us to evaluate the effect of miR-378/378* on hepatic gluconeogenesis. As expected, hepatic overexpression of miR-378/378* significantly increased gluconeogenesis in mice as indicated by the pyruvate-tolerance test (PTT) ( Fig. 1g ). In agreement with this finding, the expression levels of gluconeogenic genes, PEPCK , G6Pase and PGC-1α (peroxisome proliferator-activated receptor γ coactivator 1α), were all elevated, while the expression of small heterodimer partner ( SHP ), an inhibitor of gluconeogenesis, was decreased in the liver of mice overexpressing miR-378/378* ( Fig. 1h ). The positive regulation of gluconeogenic genes by Ad-378 was further confirmed in primary hepatocytes ( Fig. 1i ). This in vitro result also indicated that hepatic miR-378/378* regulates gluconeogenesis in a cell-autonomous manner. We also examined the glycogen storage in the liver of mice overexpressing miR-378/378*. Periodic acid-Schiff (PAS) staining result suggested that the amount of glycogen was decreased in the liver overexpressing miR-378/378* ( Fig. 1j ). Consistently, the glycogen content analysis with a glycogen assay kit showed that the glycogen level was decreased by >40% after Ad-378 infection ( Fig. 1k ). These data indicated that miR-378/378* also controls glycogen metabolism in the liver. Hepatic miR-378/378* modulates lipid metabolism Besides the abnormal glucose metabolism, we also observed a significant change of lipid metabolism in the liver after overexpressing miR-378/378*. Ad-378 infection (1 × 10 9 PFU) did not change the body weight or food intake, but resulted in a marked reduction in liver weight, hepatic triglyceride (TG) content, as well as serum TG level under feeding condition ( Fig. 1l,m and Supplementary Fig. 1g–i ). The observed alteration in hepatic TG content was further confirmed by Oil-red O staining experiment ( Fig. 1n ). Consistent with the reduced liver weight and decreased hepatic TG levels, the messenger RNA levels of lipogenic genes, ACC1 , FASN , stearoyl-CoA Desaturase 1 ( SCD1 ) and glucokinase ( GCK ), as well as the protein levels of ACC and FASN were all decreased ( Fig. 1o,p ). The negative regulation of liopogenic programme by Ad-378 was further studied in primary hepatocytes. Consistent with the in vivo results, the mRNA levels of ACC1 , FASN and SCD1 , as well as the protein levels of ACC and FASN were all decreased in primary hepatocytes on overexpressing miR-378/378* ( Supplementary Fig. 1j,k ). Thus, hepatic miR-378/378* regulates lipogenesis in a cell-autonomous manner. Hepatic miR-378/378* controls insulin signalling To understand the molecular mechanism underlying the effect of hepatic miR-378/378* overexpression on glucose homeostasis and lipid metabolism, we then investigated insulin signalling. As shown in Fig. 2a , the insulin-induced phosphorylation of Akt (S473/T308), FOXO1 and GSK3β was decreased in the liver of mice after 1 × 10 9 PFU of Ad-378 infection compared with that in control mice infected with Ad-null, indicating impaired insulin signalling. Similar results were obtained when these mice were subjected to a fasting–refeeding protocol ( Fig. 2b ). Consistent with these results, under a refed state, the mRNA levels of lipogenic ACC1 , FASN , SCD1 and GCK were lower, while the mRNA levels of gluconeogenic G6Pase , PEPCK and PGC-1α were higher in the liver of mice overexpressing miR-378/378* ( Supplementary Fig. 2a,b ). In primary hepatocytes, the insulin-induced phosphorylation of Akt was also inhibited by miR-378/378* overexpression, which was associated with relative higher expression levels of gluconeogenic G6Pase and PEPCK ( Fig. 2c and Supplementary Fig. 2c ). The translocation of FOXO1 is known to be controlled by insulin-induced phosphorylation. Thus, we analysed the effect of miR-378/378* on the cellular distribution of FOXO1. Consistent with the effect on insulin signalling, the adenovirus-mediated overexpression of miR-378/378* in primary hepatocytes significantly blocked the translocation of FOXO1 to cytoplasm induced by insulin, which resulted in nuclear accumulation of FOXO1 ( Fig. 2d,e ). The nuclear accumulation of FOXO1 was also observed in the liver of mice overexpressing miR-378/378* ( Fig. 2f ). These results further demonstrated that miR-378/378* is a potent regulator of hepatic insulin signalling. 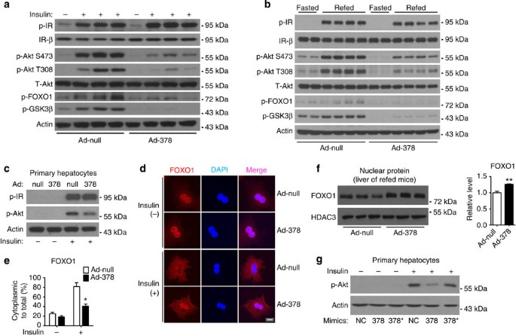Figure 2: Hepatic overexpression of miR-378/378* impairs insulin signalling. Western blot analysis of phosphorylated key molecules of insulin/PI3K pathway in the liver of mice infected with Ad-null or Ad-378 (1 × 109PFU per mouse) after insulin administration (a,n=4–8) or during the fasting-refeeding transition (b,n=5–7). (c) Western blot analysis of phospho-Akt in insulin-stimulated primary hepatocytes infected with Ad-null or Ad-378. (d) Insulin-induced endogenous FoxO1 translocation was visualized using confocal microscopy. Scale bar, 20 μm. (e) Confocal microscopy data were analysed to quantify the ratio of cytoplasmic FOXO1 to total FOXO1 in primary hepatocytes, with or without insulin treatment (n=3). (f) The level of nuclear FOXO1 in the liver of refed mice infected with Ad-null or Ad-378 (1 × 109PFU per mouse) was determined by western blot analysis and quantified. (g) Insulin-stimulated phosphorylation of Akt was analysed in mouse primary hepatocytes transfected with synthetic miRNA mimics for miR-378 or miR-378*. All experiments were repeated at least twice and representative results are shown. Figure 2: Hepatic overexpression of miR-378/378* impairs insulin signalling. Western blot analysis of phosphorylated key molecules of insulin/PI3K pathway in the liver of mice infected with Ad-null or Ad-378 (1 × 10 9 PFU per mouse) after insulin administration ( a , n =4–8) or during the fasting-refeeding transition ( b , n =5–7). ( c ) Western blot analysis of phospho-Akt in insulin-stimulated primary hepatocytes infected with Ad-null or Ad-378. ( d ) Insulin-induced endogenous FoxO1 translocation was visualized using confocal microscopy. Scale bar, 20 μm. ( e ) Confocal microscopy data were analysed to quantify the ratio of cytoplasmic FOXO1 to total FOXO1 in primary hepatocytes, with or without insulin treatment ( n =3). ( f ) The level of nuclear FOXO1 in the liver of refed mice infected with Ad-null or Ad-378 (1 × 10 9 PFU per mouse) was determined by western blot analysis and quantified. ( g ) Insulin-stimulated phosphorylation of Akt was analysed in mouse primary hepatocytes transfected with synthetic miRNA mimics for miR-378 or miR-378*. All experiments were repeated at least twice and representative results are shown. Full size image It is of interest to note that the phosphorylation levels of key components (Akt, FOXO1 and GSK3β) in insulin signalling were already decreased by miR-378/378* overexpression before insulin treatment or refeeding ( Fig. 2a,b ). Similarly, the suppression of lipogenic gene expression and activation of gluconeogenic gene expression by miR-378/378* overexpression were observed in the liver of mice under a fasted state or in hepatocytes before insulin treatment, although some of them did not reach statistical significance ( Supplementary Fig. 2a–c ). These data suggested that the basal insulin action was inhibited by miR-378/378*. To distinguish which miRNA, miR-378 or miR-378* was responsible for the suppressive effect of Ad-378 on insulin signalling, we generated synthetic mimics for miR-378 and miR-378*. We observed that only miR-378 mimics exhibited suppressive effect on insulin-induced Akt phosphorylation ( Fig. 2g ). In agreement with this finding, synthetic antagomir specific for miR-378 (Ant-378), which could reduce miR-378 level dramatically ( Supplementary Fig. 2d–f ), was able to increase the expression of lipogenic genes, such as ACC1 , FASN and SCD1 , in primary hepatocytes ( Supplementary Fig. 2e ). In addition, Ant-378 decreased the mRNA expression of G6Pase and PEPCK , and increased the mRNA expression of SHP in primary hepatocytes ( Supplementary Fig. 2f ). Based on these data, we proposed that miR-378 but not miR-378* is a regulator of hepatic insulin signalling. Metabolic effect of moderate overexpression of miR-378/378* To rule out the possibility that the observed phenotype are artefacts due to the non-physiologically high miR-378 levels following Ad-378 administration, ten times less Ad-378 (1 × 10 8 PFU) was used for in vivo experiments. As shown in Fig. 3a , miR-378 and miR-378* expression levels were moderately elevated in the liver of mice after Ad-378 infection. Similar to the observation shown in Fig. 1c,l , the glucose levels increased and the liver weights decreased in the mice with moderate overexpression of hepatic miR-378/378* ( Fig. 3b,c ). Moreover, we observed that the random glucose levels increased gradually, which is similar to the result shown in Fig. 1b , while the liver weights also decreased gradually after low-dose Ad-378 infection ( Fig. 3d,e ). Consistent with results in Fig. 1e,f , moderate overexpression of hepatic miR-378/378* led to impaired glucose tolerance and insulin tolerance ( Fig. 3g,h ). Moreover, moderately elevated miR-378/378* expression resulted in enhanced expression of gluconeogenic genes and reduced expression of lipogenic genes ( Fig. 3i–k ). These results indicated that moderate overexpression of miR-378/378* in the liver of mice is enough to affect the glucose and lipid metabolism. Furthermore, we observed that moderate overexpression of miR-378/378* in the liver of mice also has the capacity to inhibit the insulin-induced phosphorylation of Akt ( Fig. 3l ), which is similar to the result shown in Fig. 2a , further supporting the notion that miR-378/378* is an important regulator for insulin signalling. To rule out the possibility that Ad-378 infection might alter the expression of miR-378/378* in other tissues, we determined the expression of miR-378/378* in multiple tissues. As shown in Supplementary Fig. 3a,b , Ad-378 infection caused predominant overexpression of miR-378 and miR-378* in the liver but not in other tissues. 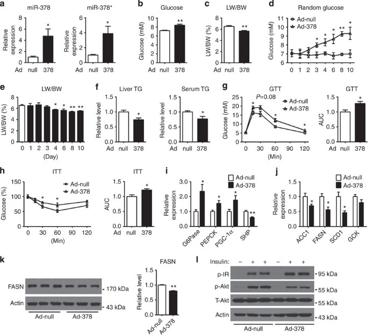Figure 3: Metabolic regulation by moderate overexpression of miR-378/378*. (a) The expression of miR-378 and miR-378* was determined in the liver of mice (n=6). Each mouse was infected with 1 × 108PFU of Ad-null or Ad-378, to achieve moderate overexpression of miR-378/378* in the liver. (b) Blood glucose levels of Ad-null or Ad-378-infected mice (1 × 108PFU,n=4). (c) The ratio of liver weight to body weight (LW/BW) in Ad-null or Ad-378-infected mice (1 × 108PFU,n=4). (d) Time course of random glucose levels of mice after Ad-null or Ad-378 infection (1 × 108PFU,n=3). (e) Time course of the ratio of LW/BW in mice after Ad-null or Ad-378 infection (1 × 108PFU,n=3). (f) Liver and serum TG levels in mice infected with 1 × 108PFU of Ad-null or Ad-378 (n=4). Glucose-tolerance test (GTT;g,n=7) and insulin-tolerance test (ITT;h,n=7) were performed in mice infected with 1 × 108PFU of Ad-null or Ad-378. AUC data for GTT (g) and ITT (h) were calculated, respectively. The mRNA expression ofG6Pase,PEPCK,PGC-1αandSHP(i), as well asACC1,FASN,SCD1andGCK(j) in the liver of mice receiving 1 × 108PFU of Ad-null or Ad-378 (n=4). (k) Western blot and densitometry analysis of FSAN in the liver of these mice. (l) Western blot analysis of phosphorylated Akt in the liver of mice infected with Ad-null or Ad-378 (1 × 108PFU) after insulin administration (n=3–6). Means±s.e.m. are shown for all panels. *P<0.05 versus control; **P<0.01 versus control (Student’st-test). All experiments were repeated at least twice and representative results are shown. Figure 3: Metabolic regulation by moderate overexpression of miR-378/378*. ( a ) The expression of miR-378 and miR-378* was determined in the liver of mice ( n =6). Each mouse was infected with 1 × 10 8 PFU of Ad-null or Ad-378, to achieve moderate overexpression of miR-378/378* in the liver. ( b ) Blood glucose levels of Ad-null or Ad-378-infected mice (1 × 10 8 PFU, n =4). ( c ) The ratio of liver weight to body weight (LW/BW) in Ad-null or Ad-378-infected mice (1 × 10 8 PFU, n =4). ( d ) Time course of random glucose levels of mice after Ad-null or Ad-378 infection (1 × 10 8 PFU, n =3). ( e ) Time course of the ratio of LW/BW in mice after Ad-null or Ad-378 infection (1 × 10 8 PFU, n =3). ( f ) Liver and serum TG levels in mice infected with 1 × 10 8 PFU of Ad-null or Ad-378 ( n =4). Glucose-tolerance test (GTT; g , n =7) and insulin-tolerance test (ITT; h , n =7) were performed in mice infected with 1 × 10 8 PFU of Ad-null or Ad-378. AUC data for GTT ( g ) and ITT ( h ) were calculated, respectively. The mRNA expression of G6Pase , PEPCK , PGC-1α and SHP ( i ), as well as ACC1 , FASN , SCD1 and GCK ( j ) in the liver of mice receiving 1 × 10 8 PFU of Ad-null or Ad-378 ( n =4). ( k ) Western blot and densitometry analysis of FSAN in the liver of these mice. ( l ) Western blot analysis of phosphorylated Akt in the liver of mice infected with Ad-null or Ad-378 (1 × 10 8 PFU) after insulin administration ( n =3–6). Means±s.e.m. are shown for all panels. * P <0.05 versus control; ** P <0.01 versus control (Student’s t -test). All experiments were repeated at least twice and representative results are shown. Full size image p110α mediates the metabolic action of hepatic miR-378 Given the fact that the effect of Ad-378 is evident for the phosphorylation of Akt (S473/T308), FOXO1 and GSK3β, but not for the phosphorylation of IR, we predicted a probable target of miR-378 located downstream of IR in the insulin signalling cascade ( Fig. 2a,b ). Bioinformatics analysis revealed that p110α , a key component of critical node in insulin signalling, contains a potential miRNA response element (MRE) for miR-378 in its 3′-untranslated region (3′-UTR). This MRE site is conserved in mice, humans and other species ( Supplementary Fig. 4a ). To determine whether p110α is a direct target gene of miR-378, the mouse p110α -3′UTR containing the MRE sequence was cloned into a luciferase reporter ( Fig. 4a ). Reporter activity analysis showed that miR-378 mimics reduced the luciferase activity of the reporter containing mouse p110α -3′UTR in a dose-dependent manner in HEK293T cells but had no effect on the reporters with mutated p110α -3′UTR ( Fig. 4b ), suggesting that p110α is indeed an miR-378 target. Similar results were obtained when human p110α -3′UTR was investigated ( Supplementary Fig. 4b ). To determine whether miR-378 is able to inhibit hepatic p110α expression, p110α protein levels were analysed in the liver of mice infected with either high- or low-dose Ad-378, as well as in hepatic cell lines. As shown in Fig. 4c and Supplementary Fig. 4c , both overexpression and moderate overexpression of miR-378/378* were able to reduce the protein levels of p110α in the liver of mice. Moreover, Ad-378 could decrease the protein levels of p110α in both murine and human hepatic cell lines ( Fig. 4d and Supplementary Fig. 4d ). In support of this, inhibition of miR-378 by Ant-378 led to an increase in the protein levels of p110α in hepatocytes ( Fig. 4e ). As miR-378 level was elevated during fasting, we also examined the protein levels of p110α in mice under different feeding conditions and observed an inverse correlation between miR-378 levels and p110α protein levels ( Fig. 1a versus Fig. 4f ). These observations clearly indicated that p110α is a direct target gene of miR-378 in the liver. 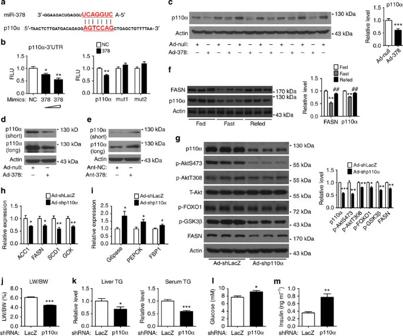Figure 4: Silencing of hepatic p110α impairs insulin signalling and metabolism. (a) Sequence alignment of the 3′-UTR of thep110αand miR-378 reveals an miR-378 response element (MRE). Seed sequences are highlighted in red. (b) The activity of the reporter containing the 3′-UTR ofp110αwas determined in HEK 293T cells in the presence of increasing amounts of miR-378 mimics (left,n=3). Reporters with two mutatedp110α-3′UTRs (mut1 and mut2) were also analysed (right,n=3). (c) Western blot and densitometry analysis of p110α protein in the liver of mice infected with 1 × 109PFU of Ad-null or Ad-378 (n=6-7). Western blot analysis of p110α in Hepa1-6 cells infected with Ad-null or Ad-378 (d), or transfected with control ant-scrambled (Ant-NC) or Ant-378 (e). (f) Western blot and densitometry analysis of hepatic p110α and FASN in fed, fasted and refed mice (n=3). Means±s.e.m. are shown. **P<0.01 (versus fed mice);##P<0.01 (versus fasted mice) (Student’st-test). (g) Western blot and densitometry analysis of key molecules in insulin/PI3K signalling, as well as p110α and FASN in the liver of mice infected with Ad-shLacZ or Ad-shp110α (n=3). (h,i) Relative expression of lipogenic genes (h,ACC1,FASN,SCD1andGCK) and gluconeogenic genes (i,G6Pase,PEPCKandFBP1) in the liver of mice infected with Ad-shLacZ or Ad-shp110α (n=7). The ratio of liver weight to body weight (LW/BW) (j), liver and serum TG levels (k), glucose level (l) and insulin level (m) were measured for the mice infected with Ad-shLacZ or Ad-shp110α (n=7). Means±s.e.m. are shown.*P<0.05, **P<0.01 and ***P<0.001 (Student’st-test). All experiments were repeated at least twice and representative results are shown. Figure 4: Silencing of hepatic p110α impairs insulin signalling and metabolism. ( a ) Sequence alignment of the 3′-UTR of the p110α and miR-378 reveals an miR-378 response element (MRE). Seed sequences are highlighted in red. ( b ) The activity of the reporter containing the 3′-UTR of p110α was determined in HEK 293T cells in the presence of increasing amounts of miR-378 mimics (left, n =3). Reporters with two mutated p110α -3′UTRs (mut1 and mut2) were also analysed (right, n =3). ( c ) Western blot and densitometry analysis of p110α protein in the liver of mice infected with 1 × 10 9 PFU of Ad-null or Ad-378 ( n =6-7). Western blot analysis of p110α in Hepa1-6 cells infected with Ad-null or Ad-378 ( d ), or transfected with control ant-scrambled (Ant-NC) or Ant-378 ( e ). ( f ) Western blot and densitometry analysis of hepatic p110α and FASN in fed, fasted and refed mice ( n =3). Means±s.e.m. are shown. ** P <0.01 (versus fed mice); ## P <0.01 (versus fasted mice) (Student’s t -test). ( g ) Western blot and densitometry analysis of key molecules in insulin/PI3K signalling, as well as p110α and FASN in the liver of mice infected with Ad-shLacZ or Ad-shp110α ( n =3). ( h , i ) Relative expression of lipogenic genes ( h , ACC1 , FASN , SCD1 and GCK ) and gluconeogenic genes ( i , G6Pase , PEPCK and FBP1 ) in the liver of mice infected with Ad-shLacZ or Ad-shp110α ( n =7). The ratio of liver weight to body weight (LW/BW) ( j ), liver and serum TG levels ( k ), glucose level ( l ) and insulin level ( m ) were measured for the mice infected with Ad-shLacZ or Ad-shp110α ( n =7). Means±s.e.m. are shown. * P <0.05, ** P <0.01 and *** P <0.001 (Student’s t -test). All experiments were repeated at least twice and representative results are shown. Full size image To determine whether p110α mediates the effect of hepatic miR-378 on glucose and lipid metabolism, as well as insulin signalling, adenovirus-mediated p110α short hairpin RNA (shRNA) was employed to knock down p110α. As shown in Fig. 4g , adenoviral p110α shRNA (Ad-shp110α) dramatically reduced the p110α protein levels in the mouse liver and, more importantly, the phosphorylation of key components of insulin signalling, including Akt (S473/T308), FOXO1 and GSK3β. Consistently, the expression levels of lipogenic genes were decreased, while the expression levels of gluconeogenic genes were increased in the liver after p110α knockdown ( Fig. 4h,i ). Similar gene expression patterns were obtained in primary hepatocytes infected with Ad-shp110α ( Supplementary Fig. 4e ). Moreover, the mice infected with Ad-shp110α exhibited normal body weight, reduced liver weight, decreased hepatic TG and serum TG levels, and elevated glucose and insulin levels, similar to the phenotype of the mice infected with Ad-378 ( Fig. 4j–m versus Fig. 1l,m and Fig. 1c,d , respectively, and Supplementary Fig. 4f,g versus Supplementary Fig. 1g,h , respectively). We also determined the protein levels of p110α in other metabolic tissues, such as inguinal fat (Ing), and muscle after Ad-shp110α infection, but only detected knockdown of p110α in the liver ( Supplementary Fig. 4h ). These data strongly suggested that hepatic p110α mediates the function of hepatic miR-378 in the regulation of insulin signalling. To test whether p110α was the only or primary target gene that is responsible for the regulatory effect of miR-378 on insulin signalling, we employed adenoviral p110α (Ad-p110α), which did not contain 3′-UTR and was supposed to be resistant to miR-378 inhibition, to restore the protein level of p110α back to a normal range in the liver of mice overexpressing miR-378/378* ( Fig. 5a ). To our greatest satisfaction, the altered glucose and insulin levels, liver weights, liver TG levels, as well as serum TG levels due to miR-378 overexpression were all corrected after the p110α protein levels were restored by Ad-p110α infection ( Fig. 5b–f and Supplementary Fig. 5a,b ). Furthermore, the effect of Ad-378 on the mRNA expression of ACC1 , FASN , SCD1 , G6Pase and PEPCK was also abolished by Ad-p110α infection ( Fig. 5g,h ). Similarly, in primary hepatocytes, after restoration of p110α expression, the suppressive effects of Ad-378 on the phosphorylation of Akt, FOXO1 and GSK3β were totally abrogated ( Fig. 5i ). These experiments clearly demonstrated that the restoration of p110α expression was able to fully rescue the phenotype of the mice and restore insulin signalling in hepatocytes infected with Ad-378. These findings suggested that the repression of p110α by Ad-378 is required for the action of miR-378 on glucose and lipid homeostasis, and hepatic insulin signalling. Based on these findings, we proposed that p110α is the primary target gene of miR-378 that mediates the action of miR-378 on hepatic insulin signalling. 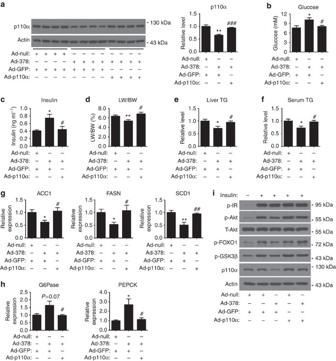Figure 5: Restoration of p110α abolishes the metabolic action of miR-378. (a) Western blot and densitometry analysis of p110α in the liver of mice infected with Ad-378 or both Ad-378 and Ad-p110α. Glucose levels (b), insulin levels (c), the ratio of liver weight to body weight (d), liver TG levels (e) and serum TG levels (f) in mice infected with Ad-378 or both Ad-378 and Ad-p110α (n=8–9). Relative mRNA expression of lipogenic genes (g,ACC1,FASNandSCD1) and gluconeogenic genes (h,G6paseandPEPCK) in the liver of mice infected with Ad-378 or both Ad-378 and Ad-p110α (n=5). (i) Western blot analysis of phosphorylated key molecules in insulin/PI3K signalling and p110α in primary hepatocytes infected with Ad-378 or Ad-p110α, or both Ad-378 and Ad-p110α after insulin administration, as indicated. Means±s.e.m. are shown. *P<0.05 and **P<0.01 (versus control group infected with Ad-null and Ad-GFP) (Student’st-test);#P<0.05 and##P<0.01 (versus the group infected with Ad-378 and Ad-GFP) (Student’st-test). All experiments were repeated twice and representative results are shown. Figure 5: Restoration of p110α abolishes the metabolic action of miR-378. ( a ) Western blot and densitometry analysis of p110α in the liver of mice infected with Ad-378 or both Ad-378 and Ad-p110α. Glucose levels ( b ), insulin levels ( c ), the ratio of liver weight to body weight ( d ), liver TG levels ( e ) and serum TG levels ( f ) in mice infected with Ad-378 or both Ad-378 and Ad-p110α ( n =8–9). Relative mRNA expression of lipogenic genes ( g , ACC1 , FASN and SCD1 ) and gluconeogenic genes ( h , G6pase and PEPCK ) in the liver of mice infected with Ad-378 or both Ad-378 and Ad-p110α ( n =5). ( i ) Western blot analysis of phosphorylated key molecules in insulin/PI3K signalling and p110α in primary hepatocytes infected with Ad-378 or Ad-p110α, or both Ad-378 and Ad-p110α after insulin administration, as indicated. Means±s.e.m. are shown. * P <0.05 and ** P <0.01 (versus control group infected with Ad-null and Ad-GFP) (Student’s t -test); # P <0.05 and ## P <0.01 (versus the group infected with Ad-378 and Ad-GFP) (Student’s t -test). All experiments were repeated twice and representative results are shown. Full size image Loss of miR-378/378* disturbs normal metabolic homeostasis To investigate the role of endogenous miR-378/378*, we took advantage of 378KO mouse model that we developed recently in our lab ( Fig. 6a and Supplementary Fig. 6a,b ). As predicted from the above findings, the protein levels of p110α were increased in the liver of 378KO mice ( Fig. 6b ). Importantly, 378KO mice exhibited increased glucose tolerance and insulin sensitivity ( Fig. 6c,d ). Moreover, both the liver weight and hepatic TG content of 378KO mice were significantly increased and the glucose levels were reduced when compared with wild-type (WT) animals ( Fig. 6e–g and Supplementary Fig. 6c ). We did not detect any alteration in body weight, serum TG levels and food intake ( Supplementary Fig. 6d–f ). Concomitant with the sensitized insulin signalling, increased hepatic content and decreased glucose levels, an increase in lipogenic gene expression and a decrease in gluconeogenic gene expression were observed in the liver of 378KO mice ( Fig. 6h,i ). These data strongly argue that increased lipogenesis and repressed gluconeogenesis due to the hepatic insulin hypersensitivity contributed to the altered glucose and lipid homeostasis in 378KO mice. 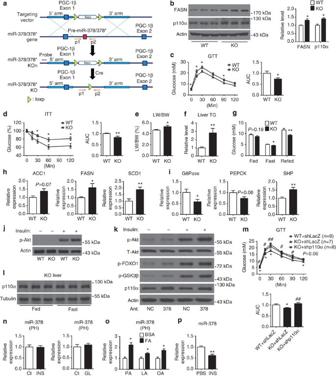Figure 6: Mice lacking miR-378/378* exhibit abnormal metabolic homeostasis. (a)miR-378gene genomic locus and targeting design. (b) Western blot and densitometry analysis of p110α and FASN in the liver of 378KO mice. Glucose-tolerance test (GTT;c,n=9–10) and insulin-tolerance test (ITT;d,n=9–10) were performed in 378KO mice. Area under the curve (AUC) data for GTT (c) and ITT (d) tests were calculated, respectively. Liver to body weight ratio (e) and liver TG levels (f) of 378KO mice (n=5). (g) Glucose levels of fed, fasted and refed 378KO mice (n=10–11). Relative mRNA expression of lipogenic genes (h,ACC1,FASandSCD1,n=5) and genes involved in gluconeogenesis (i,G6Pase,PEPCKandSHP,n=6) in 378KO mice. (j) Western blot analysis of phospho-Akt in primary hepatocytes from 378KO mice. Cells were stimulated with insulin as indicated. (k) Western blot analysis of p110α, phospho-Akt, phospho-FOXO1 and phospho-GSK3β in primary hepatocytes transfected with control ant-scrambled (Ant-NC) or Ant-378 after insulin treatment. (l) Western blot analysis of p110α in the liver of 378KO mice under different feeding conditions as indicated. (m) GTT test was performed in 378KO mice infected with Ad-shp110α or Ad-shLacZ as indicated (n=7–9). AUC data were shown (bottom). Means±s.e.m. are shown. *P<0.05 (versus WT mice infected with Ad-shLacZ);#P<0.05 and##P<0.01 (versus 378KO mice infected Ad-shLacZ) (Student’st-test). (n) Relative expression of miR-378 in primary hepatocytes treated with insulin (INS, left) or glucagon (GL, right) (n=3). (o) Relative expression of miR-378 in primary hepatocytes treated with PA, LA and OA as indicated (n=3). (p) Relative expression of miR-378 in the liver of fasted mice after insulin injection (n=3). Means±s.e.m. are shown. *P<0.05 and **P<0.01 (Student’st-test). All experiments were performed at least twice and representative results are shown. Figure 6: Mice lacking miR-378/378* exhibit abnormal metabolic homeostasis. ( a ) miR-378 gene genomic locus and targeting design. ( b ) Western blot and densitometry analysis of p110α and FASN in the liver of 378KO mice. Glucose-tolerance test (GTT; c , n =9–10) and insulin-tolerance test (ITT; d , n =9–10) were performed in 378KO mice. Area under the curve (AUC) data for GTT ( c ) and ITT ( d ) tests were calculated, respectively. Liver to body weight ratio ( e ) and liver TG levels ( f ) of 378KO mice ( n =5). ( g ) Glucose levels of fed, fasted and refed 378KO mice ( n =10–11). Relative mRNA expression of lipogenic genes ( h , ACC1 , FAS and SCD1 , n =5) and genes involved in gluconeogenesis ( i , G6Pase , PEPCK and SHP , n =6) in 378KO mice. ( j ) Western blot analysis of phospho-Akt in primary hepatocytes from 378KO mice. Cells were stimulated with insulin as indicated. ( k ) Western blot analysis of p110α, phospho-Akt, phospho-FOXO1 and phospho-GSK3β in primary hepatocytes transfected with control ant-scrambled (Ant-NC) or Ant-378 after insulin treatment. ( l ) Western blot analysis of p110α in the liver of 378KO mice under different feeding conditions as indicated. ( m ) GTT test was performed in 378KO mice infected with Ad-shp110α or Ad-shLacZ as indicated ( n =7–9). AUC data were shown (bottom). Means±s.e.m. are shown. * P <0.05 (versus WT mice infected with Ad-shLacZ); # P <0.05 and ## P <0.01 (versus 378KO mice infected Ad-shLacZ) (Student’s t -test). ( n ) Relative expression of miR-378 in primary hepatocytes treated with insulin (INS, left) or glucagon (GL, right) ( n =3). ( o ) Relative expression of miR-378 in primary hepatocytes treated with PA, LA and OA as indicated ( n =3). ( p ) Relative expression of miR-378 in the liver of fasted mice after insulin injection ( n =3). Means±s.e.m. are shown. * P <0.05 and ** P <0.01 (Student’s t -test). All experiments were performed at least twice and representative results are shown. Full size image When the hepatic insulin signalling was analysed in primary hepatocytes from 378KO mice, we observed that the phosphorylation of Akt was enhanced in hepatocytes lacking miR-378/378* ( Fig. 6j ). Moreover, the expression of gluconeogenic genes was downregulated in primary hepatocytes derived from 378KO mice, which is independent of glucagon treatment ( Supplementary Fig. 6g ). We also investigated the insulin signalling in primary hepatocytes after miR-378 level was reduced by Ant-378. Consistently, knockdown of miR-378 by Ant-378 enhanced the p110α protein levels and increased the insulin-stimulated phosphorylation of Akt ( Fig. 6k ). As the hepatic miR-378 level is transiently upregulated on fasting, one would expect that mice lacking miR378 would be able to maintain their liver p110α level without a dipping on fasting. Indeed, we found that the p110α protein expression remained unchanged on fasting in 378KO mice ( Fig. 6l ). We also investigated whether the effect of miR-378/378* was PGC-1β-dependent or whether PGC-1β expression was affected by miR-378/378* overexpression or KO. As shown in Supplementary Fig. 6h,i , both miR-378/378* deficiency and overexpression did not alter the expression of PGC-1β in the liver of mice. In addition, we also checked the expression of two known miR-378/378* targets, carnitine O -acetyltransferase ( Crat ) and mediator complex subunit 13 ( Med13 ). Consistent with the previously reported result [21] , the expression levels of both Crat and Med13 in the liver of 378KO mice on normal chow were not altered ( Supplementary Fig. 6j ). In addition to that, we did not observe significant changes in the mRNA expression levels of Crat and Med13 in the liver of mice infected with Ad-378 ( Supplementary Fig. 6k ). To further confirm the observed phenotype of the 378KO mice is hepatic p110α mediated, we inhibited p110α protein expression in the 378KO mice using Ad-shp110α. As shown in Fig. 6m and Supplementary Fig. 6l , restoration of hepatic p110α to the normal range corrected the abnormal glucose tolerance in 378KO mice. This result supported our hypothesis that hepatic p110α is responsible for the disturbed glucose homeostasis in 378KO mice. miR-378 responds to fasting and refeeding as a lipid sensor Given the ability of miR-378 to affect insulin signalling, we were interested to investigate which environmental cues or stress might regulate miR-378. As miR-378 expression level was induced during fasting and decreased after feeding, we first analysed whether glucagon is able to induce the expression of miR-378 and whether insulin acts to decrease the level of miR-378 in primary hepatocytes. We failed to observe any effect of either glucagon or insulin on the expression of miR-378 in primary hepatocytes ( Fig. 6n ). It is well known that free fatty acids (FFAs) are mobilized from fat tissues during fasting and this process is suppressed by insulin after refeeding. As it has been proposed that FFAs can mediate many metabolic effects, we speculated that miR-378 expression might be under the control of FFAs. As shown in Fig. 6o and Supplementary Fig. 6m , we observed that palmitic acid (PA), linoleic acid (LA), and oleic acid (OA) could stimulate the expression of both miR-378 and its host gene PGC-1β in mouse primary hepatocytes. This finding also suggested that miR-378 is a lipid sensor. In agreement with these findings, we found the expression of hepatic miR-378 was decreased in fasted mice after insulin injection ( Fig. 6p ). These results suggested that insulin might be able to negatively regulate hepatic miR-378 expression in vivo by controlling FFA levels via its antilipolytic effect. As miR-378 controls p110α protein level in the liver, we proposed that hepatic p110α could serve as a junction for the cross-talk between insulin signalling and fasting-responsive signalling. miR-378/378*overexpression improves steatosis in ob/ob mice Given the fact that heterozygous knockin mice carrying kinase-dead mutant p110α D933A do not exhibit abnormal glucose level, and hyperglycemia is not worsened in the ob/ob mice lacking one Akt2 allele [26] , [30] , we tested whether inhibition of hepatic p110α by miR-378 overexpression would reduce the hepatic lipid accumulation in ob/ob mice without exacerbating hyperglycemia. Interestingly, adenoviral-mediated delivery of miR-378/378* into the liver of ob/ob mice significantly reduced the liver weight and decreased the TG levels both in the liver and serum, but had no effect on fasting glucose level and body weight ( Fig. 7a–d and Supplementary Fig. 7a,b ). The reduced lipid accumulation in ob/ob mice overexpressing hepatic miR-378/378* was further confirmed by haematoxylin and eosin (H&E) and Oil-red O staining ( Fig. 7e ). As expected, hepatic p110α protein level was reduced by Ad-378 infection in ob/ob mice ( Fig. 7f ). In agreement with these findings, the mRNA expression of lipogenic ACC1 , FASN , SCD1 and GCK was decreased, while the mRNA expression of gluconeogenic PEPCK and G6Pase was not altered in ob/ob mice infected with Ad-378 ( Fig. 7g,h ). We also investigated the hepatic insulin signalling in ob/ob mice after Ad-378 infection. As shown in Fig. 7i , insulin-stimulated phosphorylation of Akt, FOXO1 and GSK3β was impaired in the liver of ob/ob mice. As we expected, the phosphorylation of Akt was further repressed by miR-378 overexpression. Consistent with the finding that Ad-378 did not alter the fasting glucose level and the expression of gluconeogenic genes ( Fig. 7d,h ), we did not observe significant effect of Ad-378 on pyruvate tolerance, glucose tolerance and insulin sensitivity in ob/ob mice by performing PTT, glucose-tolerance test and insulin-tolerance test ( Supplementary Fig. 7c–e ). These results indicated that the worsening of insulin resistance by Ad-378 is not sufficient to further exacerbate the abnormal glucose homeostasis in ob/ob mice. Collectively, these data suggested that reducing hepatic p110α level by Ad-378 might have beneficial effects on lipid metabolism without further disturbing glucose metabolism in ob/ob mice. 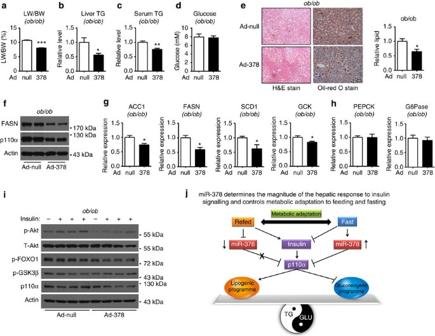Figure 7: Increasing miR-378/378* expression ameliorates steatosis inob/obmice. (a) The ratio of liver weight to body weight (LW/BW) was determined inob/obmice infected with Ad-null or Ad-378 (n=4). Liver (b) and serum (c) TG levels were measured for these mice in random fed state (n=4). (d) Fasting glucose level was also determined (n=4). (e) Representative images of H&E staining (left) and Oil-red O staining (right) of liver sections fromad libitum-fedob/obmice infected with Ad-null (top) or Ad-378 (bottom). Scale bar, 100 μm. The lipid content was quantified by Image-Pro Plus (right). (f) The protein levels of p110α and FASN. The mRNA expression of lipogenic genes (g,ACC1,FASN,SCD1andGCK) and gluconeogenic genes (h,PEPCKandG6Pase) was determined by quantitative reverse transcriptase–PCR. (i) Western blot analysis of p110α, phospho-Akt, phospho-FOXO1 and phospho-GSK3β in the liver of Ad-null or Ad-378-infectedob/obmice after insulin treatment. Means±s.e.m. are shown. *P<0.05, **P<0.01 and ***P<0.001 (Student’st-test). These experiments were performed at least twice and representative results are shown. (j) Schematic diagram of the working model of hepatic miR-378 in metabolic regulation. Figure 7: Increasing miR-378/378* expression ameliorates steatosis in ob/ob mice. ( a ) The ratio of liver weight to body weight (LW/BW) was determined in ob/ob mice infected with Ad-null or Ad-378 ( n =4). Liver ( b ) and serum ( c ) TG levels were measured for these mice in random fed state ( n =4). ( d ) Fasting glucose level was also determined ( n =4). ( e ) Representative images of H&E staining (left) and Oil-red O staining (right) of liver sections from ad libitum -fed ob/ob mice infected with Ad-null (top) or Ad-378 (bottom). Scale bar, 100 μm. The lipid content was quantified by Image-Pro Plus (right). ( f ) The protein levels of p110α and FASN. The mRNA expression of lipogenic genes ( g , ACC1 , FASN , SCD1 and GCK ) and gluconeogenic genes ( h , PEPCK and G6Pase ) was determined by quantitative reverse transcriptase–PCR. ( i ) Western blot analysis of p110α, phospho-Akt, phospho-FOXO1 and phospho-GSK3β in the liver of Ad-null or Ad-378-infected ob/ob mice after insulin treatment. Means±s.e.m. are shown. * P <0.05, ** P <0.01 and *** P <0.001 (Student’s t -test). These experiments were performed at least twice and representative results are shown. ( j ) Schematic diagram of the working model of hepatic miR-378 in metabolic regulation. Full size image Taken together, our study here demonstrated that miR-378 is a negative regulator of hepatic insulin signalling, p110α might be the primary target of miR-378 that mediates its action on insulin signalling and miR-378 regulates glucose and lipid homeostasis through suppressing hepatic insulin signalling. Based on our data here, we proposed that one of the physiological roles of hepatic miR-378 is a brake of hepatic insulin signalling. During food deprivation the brake is applied to suppress basal insulin signalling, while during nutrient excess the brake is released to sensitize insulin signalling ( Fig. 7j ). Insulin resistance predisposes an individual to the development of various metabolic diseases including type 2 diabetes. Therefore, exploring the mechanistic processes governing insulin signalling might help us to understand the pathogenesis of insulin resistance. miRNA has been shown to modulate insulin signalling directly or indirectly through epigenetic mechanisms. Identification of essential miRNAs that target critical nodes of hepatic insulin signalling will not only increase our knowledge of the molecular mechanisms underlying hepatic insulin resistance but also provide new strategies for treating metabolic disorder. Here we provided both in vivo and in vitro data to demonstrate that hepatic miR-378 is a core regulator of insulin signalling. Mice overexpressing hepatic miR-378 had elevated glucose level associated with activated hepatic gluconeogenesis and low level of hepatic TG associated with reduced lipogenic gene expression. As these mice shared many phenotypic features of liver-specific KO mice deficient in core components of insulin signalling, such as IR, p85 and p110α, we speculated that miR-378 itself might serve as a core component of hepatic insulin signalling. Indeed, we demonstrated that the p110α is a direct target of miR-378 in the liver, which would explain why the mice with hepatic miR-378 overexpression exhibited all of the hallmarks of impaired hepatic insulin signalling. In agreement with these findings, we observed enhanced insulin sensitivity, increased hepatic TG and lowered glucose levels associated with increased lipogenic gene expression and suppressed gluconeogenic gene expression in 378KO mice, strongly indicating that miR-378 is required for normal glucose and lipid homeostasis. Understanding how a specific miRNA regulates a particular biological process becomes challenging when one considers the fact that one miRNA may have hundreds or thousands of targets. Here, our data established miR-378 as a critical regulator of hepatic insulin signalling by directly targeting p110α. Knockdown of p110α in the liver of mice mimicked the effect of Ad-378. Of particular importance, restoration of hepatic p110α expression in mice infected with Ad-378 totally abrogated the action of Ad-378 on insulin signalling and insulin-controlled glucose and lipid homeostasis. Moreover, inhibition of p110α in the liver of 378KO mice corrected the abnormal glucose tolerance. These results not only suggested that the repression of p110α by miR-378 is required for the action of miR-378, but also indicated that p110α might be the only or the primary target of miR-378 that mediates all the effect of miR-378 on hepatic insulin action. FFA levels are normally at their highest in the fasting state and go down in the postprandial state due to the suppressive action of insulin on lipolysis [31] , [32] , [33] . Here we found hepatic miR-378 expression is regulated by FFA, while insulin treatment in fasted mice could reduce the expression of miR-378. Thus, we hypothesized that during fasting when insulin level is low and the suppression of FFA by insulin is attenuated, the high FFA level in turn stimulates hepatic miR-378 expression to further abrogate insulin action, to ensure that hepatic glucose production matches the whole-body requirements. In a refed state, when FFA level is decreased due to antilipolytic action of insulin on adipocytes, low FFA level leads to downregulation of miR-378, which facilitates hepatic insulin action. Thus, insulin, FFA and hepatic miR-378 form a circuit and cooperate in the regulation of glucose and lipid homeostasis. Our current study strongly supports the notion that critical nodes in insulin signalling network allow for diversification and fine-tuning of insulin signal. Insulin signalling contains three critical nodes including IR/IRS, PI3K and Akt/PKB, which are not only highly regulated but also involved in cross-talk with other signalling systems. In this study, we demonstrated that p110α catalytic subunit of PI3K is negatively regulated by miR-378 at a posttranscriptional level. Given the factor that miR-378 expression is regulated in response to fasting, we propose that p110α serves as a junction for the cross-talk between insulin signalling and fasting-responsive signalling. In this study, we showed that reducing hepatic p110α level by adenoviral miR-378/378* is able to ameliorate hepatic steatosis in ob/ob mice without exacerbating fasting hyperglycemia. This finding is consistent with previous reports showing that heterozygous knockin mice carrying kinase-dead mutant p110α D933A do not exhibit abnormal glucose level and hyperglycemia is not worsened in the ob/ob mice lacking one Akt2 allele [26] , [30] . Indeed, we observed that the insulin-induced phosphorylation of Akt was further repressed by miR-378 overexpression, suggesting that the insulin resistance was worsened. However, the impaired glucose homeostasis in ob/ob mice as manifested by glucose intolerance, insulin intolerance and pyruvate intolerance, as well as dysregulation of gluconeogenic genes, were not worsened by miR-378 overexpression. These results indicated that the worsening of insulin resistance is not sufficient to further exacerbate impaired glucose homeostasis in ob/ob mice. In summary, our study demonstrated the functional importance of hepatic miR-378 in the regulation of glucose and lipid homeostasis. Based on our findings, we proposed that hepatic miR-378 is a lipid sensor and serves as a brake on hepatic insulin signalling by directly targeting p110α, a core component of insulin/PI3K signalling ( Fig. 7j ). During fasting, increased FFAs step on the brake (miR-378) of insulin signalling to facilitate glucose production by increasing gluconeogenesis and decreasing lipogenesis. After a meal, insulin reduces the level of FFAs, which removes the brake (miR-378) to augment insulin signalling. Taken together, we proposed that miR-378 determines the magnitude of the hepatic response to insulin signalling, controls metabolic adaptation to feeding and fasting, and has therapeutic potential for hepatic steatosis. Animals All mice were males aged 8–12 weeks and were maintained on a C57BL/6J background, at a temperature of 23±3 °C and a humidity of 35±5% under a 12-h dark/light cycle (lights on at 0630, h) in a specific pathogen-free animal facility. All experimental procedures and protocols were approved by the Institutional Animal Care and Use Committee of the Institute for Nutritional Sciences, Shanghai Institutes for Biological Sciences, Chinese Academy of Science (Shanghai, China). Tissues were harvested at 1500, h without restricting the mice to food or water, unless indicated, snap-frozen in liquid nitrogen immediately after resection and stored at −80 °C. Blood samples were obtained simultaneously for serum measurements. 378KO mice were generated on a 129-genetic background at the Model Animal Research Center, Nanjing University, and were backcrossed at least six times to WT C57BL/6J mice before this study. Briefly, we used gene targeting techniques in embryonic stem cells to generate a null mutation at the murine pre-miR-378 genomic locus, which is in intron 1 of PGC-1β . The targeting vector was designed to replace pre-miR-378 gene (sequence: 5′-agg gct cct gac tcc agg tcc tgt gtg tta cct cga aat agc act gga ctt gga gtc aga agg cct-3′) of murine with a neomycin cassette. The targeted clone was identified by Southern blot analysis of EcoRV-digested embryonic stem cell DNA. After we obtained the miR-378/378* -deficient mice with neomycin (miR-378/378*KOn), we removed neomycin cassette using Cre recombination and eventually got 378KO mice. Primers used for genotyping are as follows: Mir378_loxp_tR1: 5′-CAT TGG ACA GAT GGA GAA ACA CG-3′; Mir378_loxp_tF1: 5′-GCC TCA TTT TAC AGT TGG GGA AG-3′. Heterozygous 378KO mice were mated to produce littermate WT and KO mice for study. Tolerance tests Glucose-tolerance and pyruvate-tolerance test were carried out on animals that had been fasted overnight for 16 h. After determination of fasted blood glucose levels, each animal received an intraperitoneal (i.p.) injection of 1 or 2 g kg −1 body weight of glucose or pyruvate as indicated in the figures. Blood glucose levels were detected from tail vein after 15, 30, 60 and 120 min. Insulin-tolerance tests were carried out on random-fed or 6-h fasted animals by i.p. injection of insulin (0.75 or 1 U kg −1 ) as indicated in the figures. Blood glucose levels were taken at indicated time points. Measurement of metabolic profile Glucose levels of mice were measured under different feeding condition as indicated. Liver and serum levels of triglyceride were determined according to the manufacturer’s instructions (Wako, Japan). Briefly, 50–100 mg of liver tissue was homogenized in 300 μl isopropyl alcohol and centrifuged supernatants were harvested. The extracted contents in the liver and serum were the enzymatically measured with respective kits and were expressed relative to liver weight or serum volume. The serum levels of insulin were measured by ELISA kit (Millipore, USA). Total glycogen in the liver was measured according to the methods of Glycogen Assay Kit (BioVision). Liver histology Liver-tissue H&E and Oil-red O staining were carried out after the tissues were fixed in methanol-free 4% paraformaldehyde for 24–36 h. For H&E staining, the paraffin-embedded specimens were sectioned at 5 μm and then stained. For Oil-red O staining, the subset of fixed livers were sequential 10% and 20% sucrose equilibration for 12 h each at 4 °C, and then cryoembedded in optimal cutting temperature medium. Twenty-micrometre-thick cryostat sections were prepared and stained for lipids with Oil-red O. Oil-red O staining images were taken using a light microscope (Olympus) and then quantified using Image Pro plus software (version 6.0) with colour cube-based selection criteria to ensure that only stained regions were counted, as described previously [34] . For PAS staining, the livers were harvested and fixed in absolute ethyl alcohol for 36 h and then embedded in paraffin, and 5-μm liver sections were obtained and stained for PAS staining. Primary mouse hepatocyte isolation and culture C57BL/6J mice at 8–12 weeks of age were anaesthetized with sodium pentobarbital (30 mg kg −1 i.p.) and the portal vein was cannulated under aseptic conditions. The liver was perfused with 30 ml PBS buffer containing 3.8 mg EGTA and 1% HEPES at 37 °C and then digested with 30 ml 0.05% collagenase type I solution at 37 °C. The digested mouse liver was then aseptically removed to a sterile 10-cm cell culture dish containing 10 ml cold PBS and 10 ml cold DMEM medium with 10% fetal bovine serum. The isolated mouse hepatocytes, by aspirating with a large-bore pipette, were filtrated through a 70-μm cell strainer into a 50-ml centrifuge tube and centrifuged at 500 g for 5 min at 4 °C. Cells were then suspended with 20 ml DMEM medium containing 10% PBS and were added to cold 12.5 ml Percoll solution (11.25 ml Percoll and 1.25 ml 10 × Hank’s balanced salt solution buffer) (Life Technologies). After inverting the tubes five times to ensure homogeneous suspension and centrifugation at 1,000 g for 10 min at 4 °C, the supernatant cells were removed and centrifugated cells were washed with PBS and counted. The isolated mouse hepatocytes were then cultured at 5 × 10 5 cells per well in DMEM medium containing 10% fetal bovine serum in rat-tail collagen type I-coated six-well plates overnight, before the infection with adenoviruses at a multiplicity of infection of 10. Twenty-four hours post infection, cells were maintained in serum-free DMEM containing 5.5 mM glucose overnight and treated with insulin before RNA or protein extraction. Regarding FFA treatment, PA, LA and OA were all obtained from Sigma. PA was dissolved in isopropanol at a concentration of 40 mM LA and OA were dissolved in ethanol as 100 mM stock solutions. The final treatment concentrations were all 200 μM. Before fatty acid treatment, primary hepatocytes were fasted overnight in DMEM medium containing 0.5% BSA and then treated for 4 h before RNA isolation. Adenoviruses recombination and administration The recombinant adenoviruses used for the overexpression of miR-378/378* and knockdown of p110α expression, Ad-miR-378/378* and Ad-shp110α, were generated using the BLOCK-iT Adenoviral RNAi Expression System (Invitrogen, Carlsbad, CA) in 293A cells, according to manufacturer’s instructions. Briefly, DNA fragments encoding miR-378/378* and shRNA directed against the p110α gene, respectively, were introduced into pENTR/U6 vector under the control of the human U6 promoter. The recombinant adenoviruses for p110α overexpression were generated using the AdEasy Adenoviral Vector System (Stratagene) in 293A cells. Briefly, complementary DNA encoding human p110α was cloned to pShuttle-CMV, and then pShuttle-p110α was recombined into the pAd-Easy1 vector. High-titre stocks of amplified recombinant adenoviruses were purified by two-step ultracentrifugation in caesium chloride gradient. After subsequent dialysis, viral titres were determined by the tissue culture infectious dose 50 method using 293A cells. Viruses were administered to mice through tail vein injection, using ~1 × 10 8 PFU for moderate overexpression or 1 × 10 9 PFU for overexpression in 0.25 ml PBS. Injection of the three viruses above or control viruses did not affect food consumption compared with that of control-treated animals. Mice were killed 10 days after the adenovirus injection. For infection of primary hepatocytes, viruses were used at a multiplicity of infection of 10. Quantitative PCR and northern blot analysis Total RNA of cells or tissues were extracted using Trizol reagent (Invitrogen), according to the manufacturer’s protocol. Real-time reverse transcriptase–PCR was performed as described before, with modification [35] . After reverse transcription by using PrimeScript RT reagent Kit (TaKaRa), cDNAs were quantified in ABI Real-Time System (Applied Biosystems). For miRNA detection, total RNA was reverse-transcribed using a miR-378- or miR-378*-specific stem-loop primer (Applied Biosystems) and subsequently measured by real-time PCR using miR-378- or miR-378*-specific primer (Applied Biosystems). U6 was similarly measured and used for normalization of miR-378/378* expression. Relative gene expression levels were calculated using the dd-Ct method (with U6 or TBP used as the reference gene) and normalized as indicated. The information of primers, including those for cloning, are all listed in Supplementary Table 1 . Northern blotting was performed as described previously [36] . Briefly, RNA samples were run on 15% acrylamide denaturing (urea) gels and then transferred to Nylon Positively Charged Membranes by semi-dry electrophoresis. Cross-link and hybridization was performed according to a standard protocol. 32 P-labelled DNA antisense probes complementary to mature miR-378 or 5s were used in the hybridization. miR-378 probe: 5′-CCT TCT GAC TCC AAG TCC AGT-3′; 5s probe: 5′-CAG GCC CGA CCC TGC TTA GCT TCC GAG ATC-3′. Western immunoblotting and antibodies Western blot analysis was performed as described before, with modification [37] . For the western blotting of the total lysates, we lysed tissues or cells in RIPA buffer supplemented with phosphatase and protease inhibitors. For nuclear lysates, liver tissues were extracted using NE-PER Nuclear and Cytoplasmic Extraction Reagents (Pierce), according to the manufacturer’s instruction. The lysates were subjected to immunoblotting, resolved on SDS–PAGE, transferred onto nitrocellulose membranes and probed with the various antibodies. Detection was performed by measuring the chemiluminescent signal as assayed by SuperSignal Ultra. Protein quantification was performed by Quantity One software (Bio-Rad) and the intensity values were normalized to actin or tubulin. Antibodies for IRβ, p-IR (Tyr1150/1151), Akt, p-Akt (Ser473 or Thr308), Foxo1, p-Foxo1 (Thr24)/Foxo3a (Thr32), p110α and ACC (Cell Signaling Technology, 1:1,000), p-GSK3β (Ser9) (Cell Signaling Technology, 1:3,000), FASN (BD Pharmingen, 1:3,000), HDAC3 (Santa Cruz, 1:3,000), PGC-1β (Santa Cruz, 1:500), α-Tubulin and actin (Sigma, 1:5,000) were used for blotting. Insulin signalling analysis Mice were fasted overnight for 16 h and injected i.p. with 0.75 U kg −1 of human insulin (Lilly) or saline; 10 min after injection, mice were killed and samples of liver were snap-frozen in liquid nitrogen and proteins extracted for immunoblot analysis. Mice primary hepatocytes infected with adenovirus for 36 h were serum fasted for 12 h and treated with 100 nM insulin for 5–20 min, as indicated in the figures, and cells were then harvested for reverse transcriptase–PCR, western blotting or confocal microscopy. Luciferase reporter assay Luciferase assay was performed as described before, with modification [38] . For p110α 3′-UTR-Renilla luciferase reporter assay, pRL-TK-p110α 3′-UTR reporter construct was co-transfected into 293T cells (ATCC) together with firefly luciferase plasmid pGL3 and miR-378 mimics, or Ctrl RNA (Ambion). Cells were harvested 48 h after transfection. Luciferase activity was measured using the Dual luciferase Reporter Assay System (Promega) and normalized to respective controls. Mutations in the 3′-UTR of p110α were generated with KOD-PLUS mutagenesis kit (Toyobo), resulting in altered binding sites for miR-378 as indicated, mut1site: 5′-AGUC C AG-3′ to 5′-AGUC G AG-3′ and mut 2 sites: 5′-AGU CC AG-3′ to 5′-AGU GG AG-3′. Statistical analyses Sample size was determined based on power analysis and standard practice. No data were excluded. Randomization and blinding strategy was used whenever possible. Results are expressed as mean±s.e.m. of at least three independent experiments. Statistical significance was assessed by Student’s t -test. Differences were considered statistically significant at P <0.05. The software used are Excel and GraphPad Prism 5.0 (GraphPad, San Diego, CA). NIH Image J was employed for densitometry analysis of western blotting. How to cite this article: Liu, W. et al. Hepatic miR-378 targets p110α and controls glucose and lipid homeostasis by modulating hepatic insulin signalling. Nat. Commun. 5:5684 doi: 10.1038/ncomms6684 (2014).